In-situultra-sensitive infrared absorption spectroscopy of biomolecule interactions in real time with plasmonic nanoantennas Infrared absorption spectroscopy is a powerful biochemical analysis tool as it extracts detailed molecular structural information in a label-free fashion. Its molecular specificity renders the technique sensitive to the subtle conformational changes exhibited by proteins in response to a variety of stimuli. Yet, sensitivity limitations and the extremely strong absorption bands of liquid water severely limit infrared spectroscopy in performing kinetic measurements in biomolecules’ native, aqueous environments. Here we demonstrate a plasmonic chip-based technology that overcomes these challenges, enabling the in-situ monitoring of protein and nanoparticle interactions at high sensitivity in real time, even allowing the observation of minute volumes of water displacement during binding events. Our approach leverages the plasmonic enhancement of absorption bands in conjunction with a non-classical form of internal reflection. These features not only expand the reach of infrared spectroscopy to a new class of biological interactions but also additionally enable a unique chip-based technology. Infrared absorption spectroscopy directly probes the vibrational modes associated with the various molecular bonds in a sample by measuring absorption in the mid-infrared spectral region, ~3–20 μm (3,000–600 cm −1 ) (ref. 1 ). As such, infrared spectroscopy measurements are intrinsically endowed with a level of chemical specificity and information content far exceeding most other optical measurement techniques. Fluorescence-based measurements rely on an exogenous label for their signal, while refractive index (RI) sensors [2] , [3] , [4] essentially monitor a secondary, non-specific bulk property, mass accumulation. In contrast, signal in infrared spectroscopy originates with the most intrinsic part of a sample—its molecular structure. Infrared measurements can thus be leveraged for automated tissue classification and cancer identification [5] , [6] , [7] , [8] . Most significant is their ability to record the conformational changes of proteins that elucidate the molecular mechanisms of their function [9] , [10] , [11] , [12] . Critically, such measurements do not involve any transfer of mass and are therefore largely inaccessible to other methods. Despite such advantages, several shortcomings severely limit the application of infrared absorption spectroscopy in the measurement of biological samples and their dynamic behaviour in real time. These are concerned with sensitivity and difficulties in sampling in aqueous solutions. Sensitivity is limited as a result of Beer’s law, which implies that for the small infrared absorption cross-sections, in thin samples such as monolayers, absorption signals become prohibitively weak [13] . For measurement in solution, water, though an essential component of most biological processes, presents the major obstacle. Specifically, its OH-bending absorption can overwhelm any signal from protein samples. Therefore, special care to limit path lengths to <10 μm and protein concentrations of several tens of mg ml −1 are needed to obtain the high signal-to-noise (SNR) level data required for functional studies when measurements are performed in solution [10] , [11] , [12] . This second issue is addressed in part by attenuated total internal reflection (ATR) sampling, which achieves a fixed path length via the evanescent field used to probe the sample [14] . Yet, without any signal amplification it cannot achieve adequate sensitivity. This fundamental limitation can be overcome by leveraging the strong light-matter interaction and sub-wavelength localization enabled by the plasmonic resonances of nano-scale metallic particles [15] , resulting in the phenomena of surface-enhanced infrared absorption (SEIRA) [13] , [16] , in analogy with surface-enhanced Raman scattering (SERS) [17] . Although early SEIRA studies utilized metal island films [13] , [16] , [18] , [19] , [20] , [21] , [22] , prepared by, for example, chemical means or physical vapour deposition, these are stochastic in nature, provided limited enhancement and suffered from significant repeatability issues [23] , [24] . In contrast, recent work has shown that explicitly engineered plasmonic nanoatennas with mid-infrared resonance offer reliable, 10 4 –10 5 -fold enhancement, occurring at well-defined deterministic locations [25] , [26] , [27] , [28] , [29] , [30] . To date, however, all such resonant SEIRA measurements have been performed on dry samples in either transmission or external reflection geometries. In this work, we propose and demonstrate, for the first time, that this dramatic enhancement can be applied to monitor biological samples in their native aqueous environment. We monitor protein-binding interactions via their specific amide band absorption. Signal levels measured on monolayers (175 ng cm −2 surface concentrations) correspond to a surface-averaged enhancement of a full order of magnitude over ATR, enabling high SNR measurements. Highlighting the exquisite chemical sensitivity of infrared spectroscopy, we also perform measurements on chemically distinct particles. Here we are able to chart the movement of various molecular groups, down to the displacement of minute volumes of water. Uniquely, our plasmonic system is also a chip-based technology that far exceeds ATR in terms of its compact nature and versatility. This is achieved by exploiting our nanoantennas not only to provide the aforementioned absorption enhancement but also to efficiently re-direct far-field radiation. Internal reflectance is thus provided here not by classical total internal reflection but instead by an infinitesimally thin-patterned plasmonic surface. This represents a dramatic and transformative advancement in the compatibility of infrared absorption spectroscopy with modern sample preparation and handling technologies (such as microfluidics, optical trapping and high-throughput scanning), as well as complementary optical measurement techniques. Plasmonic internal reflection-SEIRA concept The concept of our plasmonic internal reflection (PIR) technique is detailed in Fig. 1 . The basis for the chemical sensitivity of infrared spectroscopy as well as the obstacle presented by water for measuring in solution is illustrated in Fig. 1a , which shows the two major protein backbone bands, as well as the OH-bending mode. ATR overcomes this issue by probing the sample through the evanescent field associated with the total internal reflection process ( Fig. 1c ). 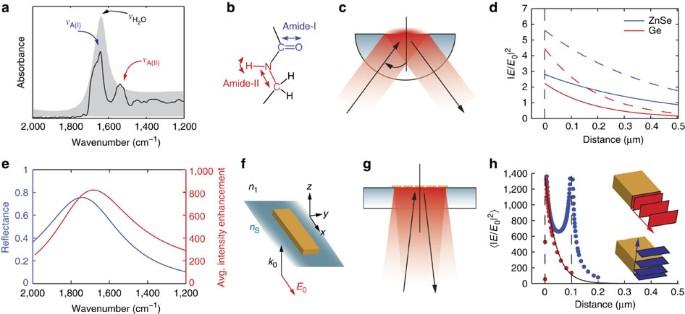Figure 1: Concept of PIR-SEIRA spectroscopy. (a) Molecular bond-specific infrared absorption spectra of protein (solid line) and liquid water (grey region). The protein backbone vibrations, amide-I and II are indicated (νA(I)andνA(II)) along with the H2O-bending mode (). (b) Molecular structure of the amide bond and associated vibrational modes (arrows). (c) Geometry of a typical single-pass ATR sampling technique. (d) E-field intensity in the sampling region with RIn=1.3. Calculations are shown forsandppolarizations (solid and dashed lines, respectively) and two different ATR crystal materials: ZnSe (n=2.4) and Ge (n=4.0). Light is incident at 45°. (e) FDTD-simulated infrared spectra of a resonant plasmonic antenna on CaF2, and (f) corresponding simulation geometry. Antennas are 1.8 μm long, 200 nm wide and 100 nm thick and are arranged in a square (P=2.5 μm period) lattice. The substrate and ambient media RIs arenS=1.4 andn1=1.3, respectively. Reflectance and near-field enhancement are shown, where the latter corresponds the average E-field intensity over a volume defined by the end-face of the rod, extended out 10 nm. (g) Geometry for PIR sampling. Light may be incident normally, as in the FDTD simulations, or at a low angle (as in experiments). (h) Spatial profile of the enhancement in the sampling volume. Simulated E-field intensity enhancement extending out, perpendicular to the end-face of the rod (red markers, schematic) or moving in thez-direction, through it (blue markers, schematic). The region over which the latter is averaged extends out 10 nm from the end-face, as ine. Note the dramatic difference in the ordinate scale in comparison withd. Figure 1: Concept of PIR-SEIRA spectroscopy. ( a ) Molecular bond-specific infrared absorption spectra of protein (solid line) and liquid water (grey region). The protein backbone vibrations, amide-I and II are indicated ( ν A(I) and ν A(II) ) along with the H 2 O-bending mode ( ). ( b ) Molecular structure of the amide bond and associated vibrational modes (arrows). ( c ) Geometry of a typical single-pass ATR sampling technique. ( d ) E-field intensity in the sampling region with RI n =1.3. Calculations are shown for s and p polarizations (solid and dashed lines, respectively) and two different ATR crystal materials: ZnSe ( n =2.4) and Ge ( n =4.0). Light is incident at 45 ° . ( e ) FDTD-simulated infrared spectra of a resonant plasmonic antenna on CaF 2 , and ( f ) corresponding simulation geometry. Antennas are 1.8 μm long, 200 nm wide and 100 nm thick and are arranged in a square ( P =2.5 μm period) lattice. The substrate and ambient media RIs are n S =1.4 and n 1 =1.3, respectively. Reflectance and near-field enhancement are shown, where the latter corresponds the average E-field intensity over a volume defined by the end-face of the rod, extended out 10 nm. ( g ) Geometry for PIR sampling. Light may be incident normally, as in the FDTD simulations, or at a low angle (as in experiments). ( h ) Spatial profile of the enhancement in the sampling volume. Simulated E-field intensity enhancement extending out, perpendicular to the end-face of the rod (red markers, schematic) or moving in the z -direction, through it (blue markers, schematic). The region over which the latter is averaged extends out 10 nm from the end-face, as in e . Note the dramatic difference in the ordinate scale in comparison with d . Full size image Our plasmonic approach is described in Fig. 1e–h . The near-field enhancement, localization and strong far-field scattering provided by the resonances of engineered mid-infrared nanoantennas form the core elements of our method. The numerical (finite-difference time domain (FDTD)) simulations in Fig. 1e demonstrate the resonances of gold (Au) rod-shaped particles, [25] , [26] , [31] on a calcium fluoride (CaF 2 ) substrate, to offer these key properties. Notably, the value of 80% reflectance on resonance corresponds to 14 times the geometrical fraction of the unit cell’s area occupied by the particles and points to the extremely efficient capture and re-direction of the incident light by the nanoantennas. This enables a unique and highly advantageous alternative to ATR, where light incident from the substrate side excites the nanoantennas, and their strong backscattering enables internal reflectance as diagrammed in Fig. 1g . This provides the opportunity to interrogate samples at the nanoantenna surface via SEIRA spectroscopy in solution, without concern for path length, as in the ATR technique. Finally, Fig. 1h probes the spatial profile of the sampling region. The plasmonic nanoantennas confine the intensity at their tip ends. [25] , [26] Normal to the substrate (blue points) variation of the field is moderate along the end-face of the rod but decays rapidly after passing the rod thickness. Parallel to the substrate (red points), perpendicular to the rod end-face, the decay is exponential, with a characteristic penetration depth (decay length) of ~80 nm, indicating a dramatically enhanced surface selectivity. Plasmonic nanoantenna design The linear rod geometry examined in Fig. 1e–h offers not only strong enhancement but also many qualities ideal for our introduced device concept. First, their resonances ( Fig. 2a ) can readily be tuned to a vibrational mode of interest through a well-characterized linear relationship between the resonance wavelength ( λ m ) and the antenna length, L [25] , [29] , [31] . Second, they scatter strongly on resonance leading to the high reflectance critical to our PIR system. The origin of this feature can be understood by applying the temporal coupled mode theory [32] , [33] , [34] to the generalized resonator model outlined in Fig. 2b . 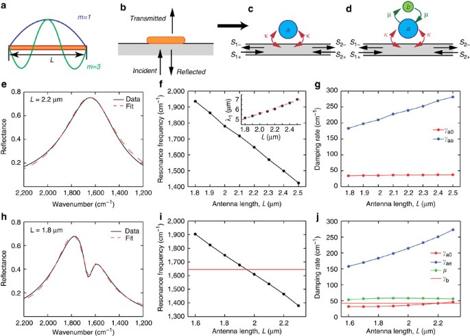Figure 2: Linear mid-infrared nanoantennas for PIR spectroscopy. (a) Physical origin of the resonances. First- (m=1) and third- (m=3) order antenna modes associated with current oscillations in rod-shaped nano-particles are illustrated. Only odd order modes couple to normally incident far-field radiation. (b,c) Generalized resonator model for the particle resonance. The resonant mode is described with amplitudeaand couples to input/output travelling waves associated with incident (s1+), reflected (s1−) and transmitted (s2−) light via the coupling constantκ. (d) Extension of the generalized resonator model to include the water OH-bend mode. This is accomplished by introducing a second resonant mode, with amplitudeb, coupled to the plasmonic resonance via μ. Three parameters: the OH-bend frequency, damping rate (νbandγb, respectively) and μ are therefore added to the model. (e–g) Simulated antenna response and extracted characteristics. Antennas are simulated as in a dry (n1=1) environment, on CaF2(nS=1.4). The width and thickness are 200 and 100 nm, respectively, andP=2.75 μm. (e) Reflectance for aL=2.2 μm antenna array and temporal coupled mode theory (TCMT) fit corresponding to them=1 resonance. (f) Variation in resonance frequency with antenna length. The inset shows the linear fit to the resonant wavelength:λ1=c1L+c0. The fit givesc1=2.63 andc0=0.37 with anr2of 0.992. (g) Radiative (γae) and non-radiative (γa0) damping rates extracted from simulated reflectance spectra as a function of nanoantenna length. (h–j) Simulated reflectance spectra, TCMT fit, extracted resonance frequencies and damping rates for nanoantennas in an aqueous environment (full complex RI of water used51). The antenna cross-section is as ine–g, while the periodicity isP=2.5 μm. In the fits,νbandγbare fixed, whereasνa,γae, γa0and μ are let to vary. (h) Reflectance spectra and fit for aL=1.8 μm antenna array (P=2.5 μm period). (i) Extracted antenna resonance frequency. (j) Extracted antenna damping rates and antenna OH-bend coupling parameter. The (fixed) values ofνbandγbare indicated by the red lines iniandj, respectively. Characterizing the antenna resonance solely in terms of its centre frequency ( ν a ), radiative and non-radiative damping rates ( γ a0 and γ ae , respectively) and coupling ( κ ) to incoming and outgoing radiation, the reflectance can be written as, Figure 2: Linear mid-infrared nanoantennas for PIR spectroscopy. ( a ) Physical origin of the resonances. First- ( m =1) and third- ( m =3) order antenna modes associated with current oscillations in rod-shaped nano-particles are illustrated. Only odd order modes couple to normally incident far-field radiation. ( b , c ) Generalized resonator model for the particle resonance. The resonant mode is described with amplitude a and couples to input/output travelling waves associated with incident ( s 1+ ), reflected ( s 1− ) and transmitted ( s 2− ) light via the coupling constant κ . ( d ) Extension of the generalized resonator model to include the water OH-bend mode. This is accomplished by introducing a second resonant mode, with amplitude b , coupled to the plasmonic resonance via μ. Three parameters: the OH-bend frequency, damping rate ( ν b and γ b , respectively) and μ are therefore added to the model. ( e – g ) Simulated antenna response and extracted characteristics. Antennas are simulated as in a dry ( n 1 =1) environment, on CaF 2 ( n S =1.4). The width and thickness are 200 and 100 nm, respectively, and P =2.75 μm. ( e ) Reflectance for a L =2.2 μm antenna array and temporal coupled mode theory (TCMT) fit corresponding to the m =1 resonance. ( f ) Variation in resonance frequency with antenna length. The inset shows the linear fit to the resonant wavelength: λ 1 = c 1 L + c 0 . The fit gives c 1 =2.63 and c 0 =0.37 with an r 2 of 0.992. ( g ) Radiative ( γ ae ) and non-radiative ( γ a0 ) damping rates extracted from simulated reflectance spectra as a function of nanoantenna length. ( h – j ) Simulated reflectance spectra, TCMT fit, extracted resonance frequencies and damping rates for nanoantennas in an aqueous environment (full complex RI of water used [51] ). The antenna cross-section is as in e – g , while the periodicity is P =2.5 μm. In the fits, ν b and γ b are fixed, whereas ν a , γ ae , γ a0 and μ are let to vary. ( h ) Reflectance spectra and fit for a L =1.8 μm antenna array ( P =2.5 μm period). ( i ) Extracted antenna resonance frequency. ( j ) Extracted antenna damping rates and antenna OH-bend coupling parameter. The (fixed) values of ν b and γ b are indicated by the red lines in i and j , respectively. Full size image where via reciprocity [32] , [33] , [34] . Equation 1 gives a Lorentzian line-shape whose amplitude and line-width are determined by the relative contributions of the loss mechanisms. In the mid-infrared, for a Drude metal such as Au, radiative damping dominates ( γ ae >> γ a0 ) and R ( ν a ) approaches unity. By fitting equation 1 to numerical simulations ( Fig. 2e ) and extracting the resonance parameters, both the linear variation in frequency ( Fig. 2f ) and dominance of radiative damping ( Fig. 2g ) are verified. The latter is an important aspect of mid-infrared plasmonics and provides the unique opportunity that PIR exploits. Although these properties depend essentially on the antenna length, periodicity in nanoparticle arrays can also influence properties [25] . Here the periodicity of the array was designed such that only the zeroth-order propagate and the unit cell size is commiserate with the antenna extinction cross-section, which optimizes the collection efficiency and ensures that equation 1 is accurate [34] . Lastly, we have extended equation 1 via the temporal coupled mode theory to include the effects of the OH-bending mode. As shown schematically in Fig. 2d , this is accomplished by introducing a coupling (via μ) between the plasmonic resonance and a purely dissipative mode with centre frequency and line-width ( ν b and γ b respectively) representative of the water absorption band. This is important because, although the calculations in Fig. 1 provided a general view of the concept and behaviour of the our PIR platform by assuming a constant and real RI, water’s absorption bands in the infrared clearly influence the response of our nanoantennas ( Fig. 2h–j ). Fitting with the analytical model therefore allows the determination of the underlying antenna parameters, which are important in validating and characterizing experimental data. In-situ sampling of protein monolayers We first demonstrate the application of PIR and the sensitivity of the technique through the measurement of a protein monolayer in dry and aqueous environments. Comparing measurements in the two allows us to characterize for the first time the effects of the overlapping water band on the enhancement and response of the nanoantennas. Our PIR chips consist of nine 100 × 100 μm 2 arrays of Au nanoantennas fabricated on CaF 2 by electron beam lithography, the dimensions being consistent with those in the simulations ( Fig. 3b ). Inserting chips into a flow cell ( Fig. 3a ) allowed measurements in aqueous environment and, in later experiments, the introduction of analyte solutions. To probe the response to a protein monolayer, the Au antennas were functionalized with a self assembled monolayer of a biotin-labelled alkanethiol (BAT) and spotted with streptavidin (SA, 50 μg ml −1 ). The specificity of the Au–thiol bond and high affinity of SA-biotin results in the formation of a ~5-nm thick SA monolayer over the Au surface. For reference, we prepared Au slides identically for measurement via grazing angle infrared reflection absorption spectroscopy (IRRAS). The absorbance spectra of one such sample is shown at the bottom of Fig. 4a (black curve). The spectra of the antennas before protein binding are shown in Fig. 4a in air and water, respectively. Extraction of the resonance parameters as in Fig. 2 yields excellent agreement with the simulations and equation 1. Measurements performed on multiple chips show excellent repeatability ( Supplementary Fig. S1 ). This highlights the practical importance of the easily controlled geometry of the nanoantennas as well as the substrate selection. The former allows highly reproducible fabrication, while CaF 2 is notable for its low RI and minimal dispersion over frequencies <1,000 cm −1 . These minimize front surface reflections that reduce throughput as well as lead to interference features. In addition, CaF 2 is transparent both in the infrared and visible region, which enables new opportunities, allowing not only easy simultaneous visible inspection of the sampling region (which we leverage here) but also the potential for, for example, parallel fluorescence detection or integration with optical trapping. 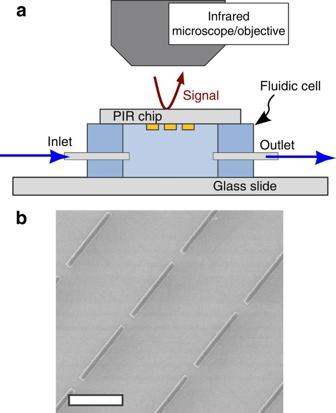Figure 3: PIR chips and experiment setup. (a) Experimental configuration for the PIR measurements (flow cell and PIR chip not to scale). (b) Representative scanning electron microscope image. Scale bar, 1 μm. The antenna array parameters are all nominally consistent with those in the numerical simulations. The cross-sectional width and thickness of 200 × 100 nm2is maintained throughout, and the periodicities areP=2.75 and 2.5 μm for dry- and aqueous-environment measurements, respectively. Figure 3: PIR chips and experiment setup. ( a ) Experimental configuration for the PIR measurements (flow cell and PIR chip not to scale). ( b ) Representative scanning electron microscope image. Scale bar, 1 μm. The antenna array parameters are all nominally consistent with those in the numerical simulations. The cross-sectional width and thickness of 200 × 100 nm 2 is maintained throughout, and the periodicities are P =2.75 and 2.5 μm for dry- and aqueous-environment measurements, respectively. 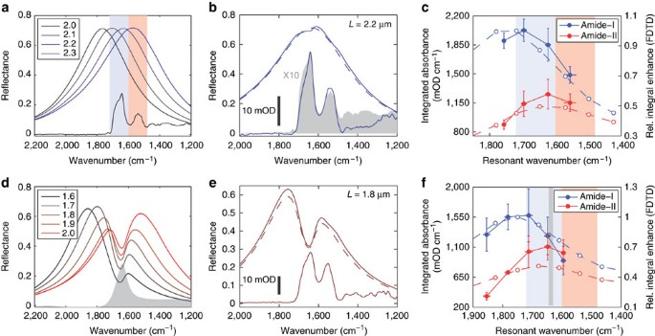Figure 4: PIR-SEIRA spectroscopy of a protein monolayer in dry and aqueous media. (a) Reflectance spectra measured for a set of nanoantenna arrays with different lengths as indicated in the legend. The spectral regions associated with the protein amide-I and II bands are indicated by the blue- and red-shaded regions, respectively. Protein spectra (taken via IRRAS) is displayed at the bottom of the figure (a.u.). (b) Reflectance spectra before (dashed) and after (solid) SA binding for theL=2.2 μm antenna array. The absorbance (see equation 2) is displayed at the bottom of the panel (solid blue line) with units indicated by the scale bar. For reference, a scaled (× 10) IRRAS absorbance spectra is displayed as the grey-shaded region. (c) Absorbance peak integral as a function of the nanoantenna resonance frequency (closed markers and solid lines; leftyaxis). Markers and error bars indicate averages and ±1 s.d. forN=3 samples. The open markers and dashed lines show the normalized FDTD-simulated intensity enhancement, scaled by relative oscillator strength of the given band (plotted against the rightyaxis). (d–e) Analogous toa–c, but for sampling in an aqueous media (data infare forN=2 samples). Ind, the grey-shaded region shows the ATR spectra of liquid water (a.u.). The grey vertical bar infindicatesfor the bending mode. Note the error bars in bothyandxin panelsc,f. The former are indicative of overall variability (which includes, for example, surface chemistry effects), whereas the latter show the variation in the plasmonic resonance, and thus point to the highly repeatable nature of infrared antenna devices by standard electron beam lithography. Full size image Figure 4: PIR-SEIRA spectroscopy of a protein monolayer in dry and aqueous media. ( a ) Reflectance spectra measured for a set of nanoantenna arrays with different lengths as indicated in the legend. The spectral regions associated with the protein amide-I and II bands are indicated by the blue- and red-shaded regions, respectively. Protein spectra (taken via IRRAS) is displayed at the bottom of the figure (a.u.). ( b ) Reflectance spectra before (dashed) and after (solid) SA binding for the L =2.2 μm antenna array. The absorbance (see equation 2) is displayed at the bottom of the panel (solid blue line) with units indicated by the scale bar. For reference, a scaled (× 10) IRRAS absorbance spectra is displayed as the grey-shaded region. ( c ) Absorbance peak integral as a function of the nanoantenna resonance frequency (closed markers and solid lines; left y axis). Markers and error bars indicate averages and ±1 s.d. for N =3 samples. The open markers and dashed lines show the normalized FDTD-simulated intensity enhancement, scaled by relative oscillator strength of the given band (plotted against the right y axis). ( d – e ) Analogous to a – c , but for sampling in an aqueous media (data in f are for N =2 samples). In d , the grey-shaded region shows the ATR spectra of liquid water (a.u.). The grey vertical bar in f indicates for the bending mode. Note the error bars in both y and x in panels c , f . The former are indicative of overall variability (which includes, for example, surface chemistry effects), whereas the latter show the variation in the plasmonic resonance, and thus point to the highly repeatable nature of infrared antenna devices by standard electron beam lithography. Full size image SEIRA spectroscopy measurements are shown in Fig. 4b . The dashed and solid blue curves show the reflectance signal after BAT functionalization and SA binding, respectively. Obvious dips associated with the amide bands are observable even in these raw spectra. The SA absorbance signal computed from the two (that is, referenced to BAT), is shown at the bottom of the figure (scale bar, 10 mOD). The curve shown has been corrected for a baseline that results from the slight red-shifting of the plasmonic resonance in response to the non-resonant, high-frequency ( n~ 1.45) component of the RI of the protein layer [25] , [35] ( Supplementary Fig. S2 ). The IRRAS-measured absorbance (multiplied by a factor of 10) is shown as the grey-shaded region. The exquisite sensitivity of the SEIRA measurement is evident, especially when one considers that a significantly smaller number of molecules and physical area are probed. Quantitatively, the peak signal for the amide-I band of 33 mOD is what would be obtained from 325 nm through a traditional Beer’s law transmission measurement. Notably, in contrast to a transmission measurement through a continuous film, the signal from our PIR sample is due to a small quantity of molecules located in the mode volume at the tips of the nano-rod antennas. Scaling for this reduced area fraction by assuming the signal to originate solely these regions, we calculate an E-field-intensity enhancement factor (EF) of 13,800. Significantly, what is actually measured in SEIRA measurements with resonant antennas is not directly absorption, but rather a perturbation of the scattering spectra resulting from coupling to a molecular resonance [29] . Resonant scattering effects have recently been examined using near-field amplitude and phase measurements [36] , indicating that the scattered signal may contain components that vary as the fourth (as opposed to second) power of the E-field [29] , [36] . Their implications are significant for our measurements, where explicitly back-scattered light is measured. This is also in accordance with the consistent observation of EFs that are either surprisingly close to or actually larger than the FDTD-simulated intensity enhancement here and in other studies [25] , [26] , [28] , [29] . Figure 4c examines the variation in this signal amplitude with the detuning of the plasmonic resonance from the frequency of the protein amide bands. Fundamentally, this explores the link between E-field enhancement and our SEIRA signal. On the practical side, this provides a measure of the bandwidth of the system and the range of frequencies that could be monitored [37] , [38] . To asses these features, the integrated absorbance over the amide-I and II bands are calculated for the four nano-rod lengths and displayed as a function of the antenna’s (far-field) resonance frequency. The data show average values and s.d. for three sets of measurements using different PIR chips and additionally point to the highly reproducible nature of the plasmonic resonances supported by our engineered nanoantennas (see especially error bars in x ). Similarly, we performed FDTD simulations for a set of different rod lengths and computed the average enhancement over a range of frequencies corresponding to a given absorption band (for example, amide-I or II). These were then scaled to account for the different intrinsic oscillator strengths associated with the two bands and normalized to a maximum value of 1. First, we observe a general correspondence between the trends for experiment and from FDTD predictions, while subtle effects such as the slightly sharper experimental curves are indicative of the aforementioned resonant scattering effects [29] , [36] . Second, both simulation and experiment point to a promising bandwidth. The plasmonic resonance can be detuned ~300 cm −1 before the signal level drops <75% of the maximum, indicating that a single antenna design could probe a fairly broad range. That similar measurements can readily be performed in solution using the PIR chip is demonstrated in Fig. 4d–f . The effect of the water vibrational band is clearly visible in the plasmonic reflectance spectra (grey-shaded region displays an ATR-measured spectrum from water for reference). Though the plasmonic substrates confine the E-field to within 80 nm of the surface, the 20% modulation in reflectance due to the water band points to the significant SEIRA enhancement. Critically, however, a 5-nm thick protein monolayer bound to the nanoantenna surface represents a far greater fraction of this path-length than it would for a traditional transmission measurement. Thus, as shown in Fig. 4e , high-quality spectra can readily be obtained for molecules in an aqueous environment. The slight reduction in signal results from the increased damping of the plasmonic resonance due to the water band, corroborated by the variations in Fig. 4f . Yet, the 22 mOD signal is still significant, corresponding to an EF of 7,700 and, significantly, over an order of magnitude increase over what would be measured via ATR sampling ( Supplementary Fig. S3 ). Finally, we emphasize the extremely high SNR evident in our measurements. Comparing the IRRAS measurement with our SEIRA spectra, the SNR are found to be comparable. This is significant, given that our PIR signal comes from only a 100 × 100 μm 2 region, which represents a 3,000-fold reduction in sample area compared with IRRAS. Further improvements in the SEIRA SNR should be straightforward, for example, by utilizing a polarization-intensive antenna. Our PIR platform thus offers significant advantages over the state of the art infrared techniques, effectively overcoming the significant complications in measuring protein monolayers in aqueous environments, while introducing a level of compactness and versatility previously absent. In-situ protein immunoassays via chemical fingerprints The ability of our PIR technology to operate in aqueous environments at high sensitivity and SNR is ideally suited to time-resolved studies of biomolecules and other chemical species at the monolayer level. We demonstrate this application by monitoring a series of biologically relevant protien–protien-binding events as well as chemically distinct model substances. The latter set of measurements is notable, given that RI sensors probe only mass accumulation and are thus incapable of performing a distinction that, as will be shown, is straightforward with our infrared measurements. We first performed three assays, each consisting of three proteins. The PIR chips were inserted into the flow cell following BAT functionalization. Spectra were recorded at 5 min intervals, as the various buffers and protein solutions were introduced. On the basis of the considerations detailed in Fig. 4f , we monitored the L =1.8 μm array throughout. The protein interactions studied are shown schematically in Fig. 5a . The three assays shown were performed in series, one after the other using different PIR chips (albeit containing nominally identical sets of plasmonic arrays). All three experiments are identical in their first two steps, which consist of SA followed by a biotin-labelled anti-rabbit (goat host) ( (b) αR(G)) IgG. For the third step, a target IgG intended to interact with the immobilized (b) αR(G) is introduced. This IgG is varied between the three experiments to provide different levels of binding. Specifically, anti-goat (mouse host) (αG(M)), rabbit IgG (from serum) (R(s)) and mouse IgG (from serum) (M(s)) were chosen to provide high, weak and zero-specific binding to the immobilized (b) αR(G). These are estimated to correspond to high- (≥1), weak- (likely ~1/3), and zero-bound target per immobilized (b) αR(G) [39] , [40] . In all experiments, for each step the protein solution is introduced at a concentration of 50 μg ml −1 and allowed to flow for 1 h. Each step is followed by a 15-min rinse with a detergent, then pure buffer. 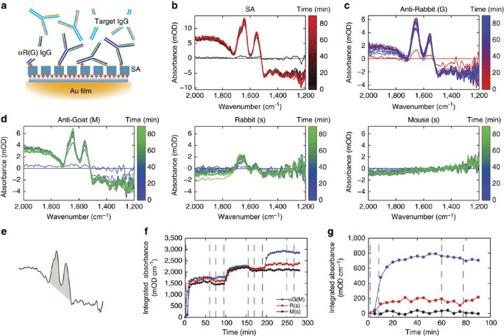Figure 5: Multiple protein binding monitoredin-situwith PIR-SEIRA. (a) Schematic of protein-binding interactions measured. (b–d) Time series of spectra taken during (b) SA, (c)(b)αR(G) and (d) three target IgG-binding steps. (e) Amide band peak integral used to asses protein binding. (f) Peak integral (integrated absorbance) evolution over time during the protein-binding measurements for the three samples. (g) Expansion of the incremental change during the three different target IgG-binding step. Figure 5: Multiple protein binding monitored in-situ with PIR-SEIRA. ( a ) Schematic of protein-binding interactions measured. ( b – d ) Time series of spectra taken during ( b ) SA, ( c ) (b) αR(G) and ( d ) three target IgG-binding steps. ( e ) Amide band peak integral used to asses protein binding. ( f ) Peak integral (integrated absorbance) evolution over time during the protein-binding measurements for the three samples. ( g ) Expansion of the incremental change during the three different target IgG-binding step. Full size image Differential absorbance spectra at each time are plotted in Fig. 5b–d . For each step, the absorption is referenced to the spectra taken immediately before the given protein solution is introduced. Each set of spectra therefore give the increase in absorption solely due to the binding of the protein associated with the given step. Because of the relatively low dielectric constant contrast between the bound protein and water (as compared to air) and the fact that we monitor a single nanoantenna array throughout, it was not necessary to perform the baseline correction used in conjunction with Fig. 4 . As a result, we observe the progression of a slowly varying step-like feature in our spectra associated with a shift in our plasmonic resonance as material binds. Focusing on the specific protein absorption bands, for the three different target IgG steps, shown in Fig. 5d , we observe significant increase in the amide band absorption for the αG(M), much smaller signals from R(s) and apparently no binding from the M(s) IgG. These observations can be summarized and displayed in a more quantitative fashion by computing the peak integrals as a function of time, as shown in Fig. 5e–g . The number of amide bonds corresponds to the number of amino acids in a protein; hence, the integral over the total amide-I and II peak region ( Fig. 5e ) serves as a proxy for protein accumulation. The resulting binding curves in Fig. 5f are qualitatively similar to those that can be obtained with RI sensors and also quantitative in nature. For the first two steps, the three experiments show excellent agreement, highlighting the high degree of repeatability of our measurements. For the target IgG step, shown in detail in Fig. 5g , the varying degrees of binding are evident, with roughly 1/3–1/4 the amount of R(s) compared with αG(M). Importantly, despite the similarity of the appearance of these results to those of label-free sensors, the signal here corresponds directly to the number of amide bonds present. It is therefore specific to the chemical structure of the bound molecules as opposed to non-specific mass accumulation. Identification and tracking of chemically distinct substances We highlight this key ability of infrared spectroscopy to measure molecular bond-specific fingerprints and demonstrate the implied capability to distinguish and track chemically distinct substances in Fig. 6 . Binding interactions as in Fig. 5 are monitored. The experiment consists of two binding steps, SA followed by biotin-labelled latex beads ( (b) LB), shown in Fig. 6a . Although both the protein and beads have similar RIs in the visible/near-infrared, their different molecular structure is immediately apparent in the spectra shown in Fig. 6b . Styrene contains no amide bonds; hence, the characteristic absorption peaks associated with the protein binding are entirely absent in the (b) LB spectra shown in Fig. 6c . Instead, two narrow bands at ~1,490 and ~1,450 cm −1 appear. These can be assigned to vibrational modes associated with the benzene ring in the styrene molecule, shown in Fig. 6d . An additional feature of note is the broad negative peak, corresponding to a reduction in absorption, at ~1,650 cm −1 . We assign this feature to the OH-bend vibration of liquid water and propose that it results from its displacement as the beads bind at the nano particle surface. Such effects are likely not observed during the protein-binding steps because of the fact that proteins are essentially highly flexible folded strands that can interact with and internalize a significant amount of water molecules. Therefore, in contrast to the beads, they can be thought of as extremely porous and do not displace water to the same degree. 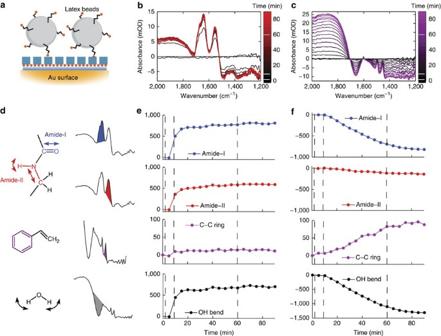Figure 6: Molecular bond-specific signatures of bound particles. (a) Schematic of the latex bead–SA binding. (b,c) Time-series absorbance spectra during the SA- and(b)LB-binding steps. (d) Specific chemical structures and their corresponding infrared fingerprints (peak integrals) used to monitor their presence during the flow experiments. (e,f) Evolution of the peak integrals (integrated absorbance, units of mOD cm−1) over time during SA- and(b)LB-binding steps, respectively. Figure 6: Molecular bond-specific signatures of bound particles. ( a ) Schematic of the latex bead–SA binding. ( b , c ) Time-series absorbance spectra during the SA- and (b) LB-binding steps. ( d ) Specific chemical structures and their corresponding infrared fingerprints (peak integrals) used to monitor their presence during the flow experiments. ( e , f ) Evolution of the peak integrals (integrated absorbance, units of mOD cm −1 ) over time during SA- and (b) LB-binding steps, respectively. Full size image The chemically distinct substances monitored here thus consist of protein, liquid water and polystyrene. The characteristic peak integrals and associated molecular vibrations are shown in Fig. 6d . Both the amide-I and II are monitored separately, as the amide-I overlaps with the OH bend, which also varies over the course of the measurements. The ability to sensitively chart the movement of the various chemical groups, as shown in Fig. 6e , adds a clear extra dimension to infrared spectroscopy with our plasmonic technique, not present in traditional label-free techniques. The ability to monitor such subtle effects as the displacement of minute quantities of water molecules further highlights the level of information that can be obtained on trace samples via PIR measurements. With the proposed PIR technique and its usage to detect and chemically identify the constituents in binding interactions, we demonstrate a highly sensitive, compact and versatile chip-based platform for in-situ infrared absorption spectroscopy. The high-quality data with large SNR imply the opportunity for detailed infrared studies down to the single-molecule level. Significantly, beyond the chemical identification capability demonstrated here, the extension of this system to monitoring conformational changes that do not result from mass accumulation, and are therefore largely invisible to RI sensors, should be possible. The ability to perform such measurements in situ on monolayer thickness samples enables studies involving direct electron transfer, such as redox reactions, as well as the investigation of important interface effects [21] , [22] . Our reliance on engineered plasmonic nanoantennas allows for highly repeatable measurements, well-defined detection volumes and large EFs, as demonstrated in Fig. 4 . Furthermore, it allows for the large body of research on plasmonic nano particle design to be put to use, to deterministically tailor resonance properties as desired for a given experiment [15] , [35] , [41] , [42] , [43] , [44] , [45] , [46] . Finally, the ability to efficiently re-direct far-field radiation in the manner implemented here is unique to engineered nanoantennas and critical to our chip-based design that eliminates the need for bulky high-index ATR crystals and their associated coupling optics. Recent work on directional plasmonic antennas can be used to optimize or find new functionalities related to this feature as well [47] , [48] , [49] , [50] . Our measurements here, performed in an infrared microscope with a single element detector, provide an initial demonstration of the capabilities and convenience of our PIR technique. Looking forward, in conjunction with improvements in infrared detectors and source technology, such as bright quantum cascade lasers, PIR enables a number of interesting new possibilities. In combining dramatic signal amplification with a non-classical internal reflectance mechanism, our platform enables infrared absorption spectroscopy to be performed on monolayer thickness samples with unparalleled sensitivity in a chip-based platform. This opens the door for both a new class of infrared absorption sensors and spectroscopy tools, as well as a new community from, for example, nano-photonics, microfluidics and other backgrounds to take advantage of their immense potential. Numerical calculations Numerical (FDTD) simulations were performed using a commercial software package (Lumerical). Periodic boundary conditions were used throughout with excitation due to a normally incident plane wave entering the simulation domain from the substrate side (see Fig. 1f ). The dielectric constants of Au and H 2 O were taken from Palik [51] . A thin (5 nm) chromium (Cr) adhesion layer, present in the fabricated samples, was omitted from the simulations. A local mesh with spacing δ =1 nm in a region about the tip ends of the rods was used. The average E-field intensity enhancement over a given frequency band (amide-I or II) was computed from FDTD simulations via , where | E / E 0 | 2 denotes a spatial average over the volume defined in Fig. 1e . Thus, F I = F (1,600 cm −1 , 1,720 cm −1 ) and F II = F (1,500 cm −1 , 1,600 cm −1 ) were obtained as functions of the nanoantenna array resonance frequency for the amide-I and II bands, respectively. To account for the different intrinsic oscillator strengths associated with the two protein bands, we scaled F II by the ratio of the amide-II- to amide-I-band-integrated absorbance obtained from the IRRAS data (for which enhancement varies negligibly with frequency). Finally, to compare the trends in the field enhancement with the experimental data, F I and the scaled F II were normalized to a maximum value of max( F I )=1 for the dry- and aqueous-environment measurement sets. Sample fabrication Samples were fabricated via electron beam lithography and lift-off on CaF 2 windows (13 mm diameter; 1 mm thick). Particles are formed by depositing a 5-nm thick Cr-adhesion layer followed by 100 nm of Au via electron beam evaporation. Following lift-off, an O 2 plasma clean was used to remove any small residual amount of poly(methyl methacrylate). Samples were stored under vacuum before use. Gold slides for IRRAS measurements were prepared in-house through evaporation of Cr/Au (identically to the particles) on polished silicon. Spectroscopic measurements FTIR measurements were performed on a Bruker IFS 66/s spectrometer using a mercury cadmium telluride detector. All data were taken under identical acquisition settings: a mirror velocity of 40 kHz, 512 scans co-added and 8 cm −1 resolution. Reflectance measurements are referenced to an Au mirror. SEIRA measurements were performed with an infrared microscope (Hyperion 1000; Bruker) with a 0.4 numerical aperture, × 15 objective. Knife edge apertures limited the collected signal to a single 100 × 100 μm 2 array for each measurement. A plastic enclosure was purged with dry and CO 2 filtered air to limit interference from water vapour lines. Typically reference water vapour spectra were recorded and used to subtract out any residual lines. Grazing angle (80 degree from the surface normal) IRRAS measurements were performed to characterize the SA protein absorbance [26] , [25] . Samples of ~1 × 1 in were used and placed on a mask that limited the sampling area to about 6 mm in diameter. Notably, because samples are also formed on Au slides, not only can identical preparation techniques be used but also the sample is probed by the E-field oriented perpendicular to the Au surface, just as in SEIRA; hence, the same component of the sample dielectric function is measured. ATR measurements were performed using a single-reflection accessory, with spectra ratioed to a background spectra recorded from the bare crystal. In addition to the IRRAS reference measurements, two sets of control measurements were performed. In the first, samples were fabricated and measured such that the nanoantenna resonances were scanned over a wide range of wavelengths and show the characteristic Fano line-shapes, and eventual decay in amplitude of the amide bands and the antenna resonances are detuned ( Supplementary Fig. S4 ). In the second, measurements were performed with light polarized perpendicular to the antenna long axis such that no resonances were excited and show, as a consequence, no amide band features ( Supplementary Fig. S5 ). Both were performed in dry and aqueous environments. For the SEIRA measurements in an aqueous environment, a small fluidic chamber was constructed out of polymethyl disiloxane. The chamber was irreversibly sealed at its bottom to a glass microscope slide by O 2 plasma oxidation and Si–OH bonding. The CaF 2 sample was pressure sealed to form the top window of the fluidic cell as shown in Fig. 3 . The volume of the chamber was approximately 0.5 ml, measured by filling with a syringe pump. For static measurements ( Fig. 4 ), the chamber was filled with PBS, and the inlet and outlets were sealed to prevent flow. During binding measurements ( Figs 5 and 6 ), a constant flow rate of 0.14 ml min −1 was maintained. Data processing and analysis Equation 1 and the modified version (including the OH-bend mode) used to extract antenna resonance parameters are derived in Supplementary Methods . The absorbance spectra used to analyse protein and biomolecule binding are determined from reflectance measurements using equation 2. The resultant spectra display absorption bands associated with the SEIRA effect as well as a step-like baseline. This baseline results from the fact that the binding of protein to the surface of the nanoantenna resonators shifts their centre frequencies, because of the n ~1.45 non-dispersive component of the protein’s RI. Although polynomial baseline correction is common in infrared spectroscopy, we used the physical origin of the feature to constrain the functional form of the fit. The specific function used and fitting procedure are included in Supplementary Methods . The SEIRA enhancement was quantified in terms of an effective path length ( d e ) [52] , EF and comparison with ATR. These all began with our IRRAS measurements, from which the expected transmission signal from an ideal Beer’s law measurement was determined via the relation The high-frequency protein RI, n ∞ =1.48, is determined from a fit (equation 4 below), and θ =80° is the incident angle in the IRRAS measurements. The 3.01 mOD for IRRAS correspond to 0.44 mOD from equation 3. For a thin film, the effective path length is then d e ≈ d (Δ R /Δ T ), where Δ R is the change in reflectance from the SEIRA measurement, and Δ T is given by equation 3 (derivation in Supplementary Methods ). The EF is the signal enhancement, scaled to account for the reduced area fraction as EF =(Δ R /Δ T )/ A , where A =2 wt / P 2 is the area fraction ( w =200 nm and t =100 nm being the nominal rod width and thickness, respectively) of the unit cell occupied by the (two) rod tips. Comparison with ATR was accomplished by calculating the expected signal for an ATR measurement from the Fresnel equations [52] ( Supplementary Fig. S3 ). Here the SA dielectric function was approximated by fitting IRRAS data with a two-oscillator dielectric function, for the amide-I and II bands. [25] For the amide-I band, the calculated absorbance for ATR was determined to be 1–1.4 and 0.4–0.7 mOD for ZnSe and Ge elements, respectively. Both show similar overall throughput ( Supplementary Fig. S3 ) to our PIR method. Peak-to-peak and root mean square noise levels were determined or both the IRRAS and SEIRA absorbance were evaluated over the standard 2,000–2,200 cm −1 mid-infrared window. [1] This noise value was scaled for the nanoantenna measurements to account for the fact that the window lies at the edge of the reflectance peak. Peak-to-peak (root mean square) values of 160 (680), 80 (310) and 110 (480) SNRs were thus determined for the dry- and aqueous-environment SEIRA and IRRAS measurements, respectively. Peak integrals comparing chemical bands’ signatures were computed via , for the amide-I, II, combined amide-I and II, H 2 O and CC regions as shown in Figs 4 , 5 , 6 . The parameter h is a reference line connecting two selected points ( ν h1 and ν h2 ), that is, h = m ( ν − ν h1 )− A k , j ( ν h1 ) where m =( A k , j ( ν h2 )− A k , j ( ν h2 ))/( ν h2 − ν h1 ) is the slope ( Supplementary Table S1 ). As the RI contrast between protein and water is small (relative to protein and air) and our binding measurements used a single plasmonic structure, the linear reference line was sufficient for analysis of the data in Figs 5 and 6 without the aforementioned constrained baseline correction. Surface chemistry and binding protocols The formation of the BAT (CMT015-25; Nanoscience Instruments) self-assembled monolayer (SAM) on our Au nanoantennas was accomplished by incubating samples in an 0.5-mM ethanol-based solution overnight. SA (21125; Pierce) was attached, either by spotting (~20 μl volume spot) and incubating for 1 h, as in the case of the static measurements ( Fig. 4 ), or by circulating the solution in a flow cell, as in the time-resolved measurements ( Figs 5 and 6 ). In either case, a 50 μg ml −1 solution in PBS was used. Spotted samples were rinsed in PBS with detergent (tween 20) (PBST) for 5 min, followed by pure PBS and Millipore water, 5 min each. The flow experiments followed a similar rinsing procedure, consisting of 15 min of PBST followed by 15 min of PBS [3] . For the immunoassays, IgG samples were selected based on their recognition and host properties ( Supplementary Methods ). All were used at concentrations of 50 μg ml −1 diluted in PBS. Given the low intensity on the sample of the Globar source used in the experiments, protein de-naturing due to thermal effects was not a concern ( Supplementary Methods ). For the bead experiments, biotin-labelled latex beads with a mean size of 250 nm were used (L7655; Sigma). The solution was diluted to 0.01% solids (weight/weight) in PBST corresponding to 1.2 × 10 10 particles per ml (50 pM). SPR measurements were performed on an immunoassay to check binding kinetics and the deposited surface density of the SA layer ( Supplementary Fig. S6 ). Measurements were performed on a Biacore 3000 using Au chips functionalized with BAT as in the FTIR measurements. A response of 1750 RU was measured for SA, corresponding to a surface concentration of ~175 ng cm −2 (1 RU=1 pg mm −2 for proteins [53] ), in close agreement with the value of ~200 ng cm −2 in Peluso et al . [39] How to cite this article: Adato, R. and Altug, H. In-situ ultra-sensitive infrared absorption spectroscopy of biomolecule interactions in real time with plasmonic nanoantennas. Nat. Commun. 4:2154 doi: 10.1038/ncomms3154 (2013).